Heterogeneity in theDrosophilagustatory receptor complexes that detect aversive compounds Animals must detect aversive compounds to survive. Bitter taste neurons express heterogeneous combinations of bitter receptors that diversify their response profiles, but this remains poorly understood. Here we describe groups of taste neurons in Drosophila that detect the same bitter compounds using unique combinations of gustatory receptors (GRs). These distinct complexes also confer responsiveness to non-overlapping sets of additional compounds. While either GR32a/GR59c/GR66a or GR22e/GR32a/GR66a heteromultimers are sufficient for lobeline, berberine, and denatonium detection, only GR22e/GR32a/GR66a responds to strychnine. Thus, despite minimal sequence-similarity, Gr22e and Gr59c show considerable but incomplete functional overlap. Since the gain- or loss-of-function of Gr22e or Gr59c alters bitter taste response profiles, we conclude a taste neuron’s specific combination of Grs determines its response profile. We suspect the heterogeneity of Gr expression in Drosophila taste neurons diversifies bitter compound detection, improving animal fitness under changing environmental conditions that present a variety of aversive compounds. Animals use their sense of taste mainly for evaluating food quality. Animals detect potentially harmful compounds in their food to avoid ingesting toxic chemicals. Many toxic compounds taste bitter and induce aversive behaviors. Since many plants defend themselves against herbivory by producing a diversity of bitter compounds, many herbivorous insects have evolved gustatory systems capable of detecting large numbers of bitter compounds. Higher concentrations of these bitter compounds elicit more robust behavioral aversion, suggesting bitter-responsive cells discriminate concentration [1] . It remains unclear, however, whether the bitter taste modality perceives a generic “bitterness” leading to a generic behavioral aversion or whether the system shows more specific molecular discernment permitting more subtle, complex behavioral responses. The bitter-responsive cells of several species reportedly express heterogeneous groups of bitter receptors [2] , [3] and they respond to distinct bitter compounds [3] , [4] , [5] . Still, the consequences of this heterogeneity of bitter receptor expression have not been fully explored at the molecular and cellular levels. Drosophila have taste organs all over the body including the labellum, legs, pharynx, anterior wing margin, and even the female genitalia [6] , [7] . Of these locations, the Drosophila labellum is an attractive place to study bitter taste receptor heterogeneity. The bitter-responsive taste neurons of the labellum are easily accessible for electrophysiological analyses, and we have many genetic reagents that permit precise control over bitter receptor expression in the bitter-responsive taste neurons. Each half-labellum contains 31 taste sensilla classified by their relative length and location into Large (L)-type, Intermediate (I)-type, and Small (S)-type [8] . According to electrophysiological analyses of these 31 taste bristles, all three types of sensilla show distinct response profiles to bitter compounds [3] . After mapping these response profiles to the various morphologic classes, it became clear that the labellar taste sensilla should actually be divided into five classes (Fig. 1a ) [3] . L-type and S-c sensilla show almost no response to bitter compounds. S-a and S-b sensilla are broadly tuned, with S-b sensilla showing robust responses to most bitter compounds. I-a and I-b sensilla are narrowly tuned, with complementary response profiles to bitter compounds [3] . Fig. 1 Identification of Grs for LOB, BER, and DEN detection. a Spatial localization of each class of taste bristle in the labellum. Figure modified from Weiss et al. [3] (2011). b Schematic for the misexpression of bitter Grs from I-a sensilla in the sweet GRNs of L-type sensilla using Gr64f - GAL4 . The Grs normally expressed in bitter GRNs of I-a sensilla and their bitter ligands (red), as well as the sweet Grs normally expressed in sweet GRNs of L-type sensilla and their sugar ligands (blue) are indicated. c Representative traces from L-type sensilla of flies of the indicated genotypes upon application of 1 mM stimuli of LOB, BER, or DEN. d Mean responses of L-type sensilla induced by the indicated chemicals: 100 mM sucrose (SUC), 1 mM LOB, 1 mM BER, 1 mM DEN, 5 mM CAF, 1 mM STR, 1 mM SOA, and 1 mM UMB. n = 6–10. Unpaired t -test or the Mann−Whitney U -tests as appropriate. e Identification of the Grs required for LOB, BER, and DEN detection. The mean responses of L-type sensilla of the indicated genotypes upon application of 1 mM stimuli of LOB, BER, and DEN as well as 100 mM SUC are shown. n = 6–10. ANOVAs followed by Dunnet T3 post hoc tests for LOB and the Kruskal−Wallis tests followed by Mann−Whitney U post hoc tests for BER and DEN. The asterisks indicate statistically significant differences from Gr64f >6 Gr s flies in d . f The mean responses of L-type sensilla expressing Gr32a , Gr59c , and Gr66a induced by the indicated chemicals. n = 6–10. Unpaired Student’s t -tests or the Mann−Whitney U -tests as appropriate. All data are presented as means ± S.E.M. * p < 0.05, ** p < 0.01. Complete genotypes are listed in Supplementary Table 6 Full size image Several classes of chemosensory receptors have been suggested as taste receptors for the detection of aversive chemicals [9] , [10] , [11] , but most bitter compound detection requires members of the gustatory receptor (GR) family. The 60 Gr genes in the fly genome encode 68 proteins by alternative splicing [12] , [13] . The bitter gustatory receptor neurons (GRNs) of each sensilla class (i.e., S-a, S-b, I-a, and I-b) express distinct Gr subsets [3] . For example, while bitter GRNs in S-a sensilla co-express 29 bitter Grs , bitter GRNs in I-a sensilla express a combination of 6 bitter Grs . The role the Grs play in taste has been extensively studied by in vivo loss-of-function [14] , [15] , [16] , [17] , [18] , [19] , [20] , but those experiments have limitations. 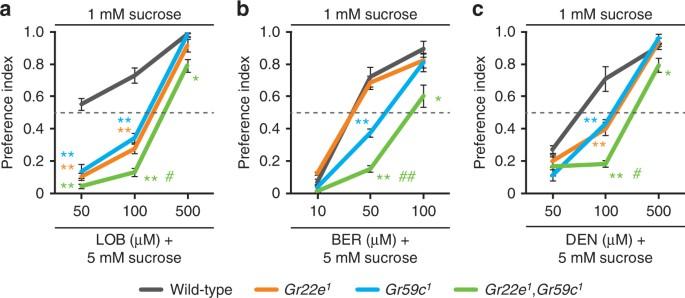Fig. 6 The contribution ofGr22eandGr59cto bitter food aversion. Two-way choice assays using the indicated concentrations ofaLOB,bBER, andcDEN.n= 4–12. ANOVAs followed by Tukey post hoc tests or Kruskal−Wallis tests followed by Mann−Whitney U post hoc tests as appropriate. All data are presented as means ± S.E.M. The asterisks and sharps indicate statistically significant differences from wild-type flies (*p< 0.05, **p< 0.01) and from bothGr22e1andGr59c1(#p< 0.05,##p< 0.01), respectively Most of those studies focused on flies carrying mutations in individual Grs , measuring the bitter response profiles of very limited numbers of sensilla. Since bitter GRN response profile and Gr expression profile are different depending on sensilla type and since multiple independent GRs are required for bitter compound detection [20] , it seems reasonable to assume the function of a given Gr depends on the Grs with which it is co-expressed. Indeed, in vivo misexpression of an individual Gr in different bitter GRNs induces differential effects, likely due to the other Grs they express [21] . Still, the precise molecular and cellular role Grs play in the detection of aversive chemicals remains unclear. In this study, we attempt to parse the function of the bitter Grs in Drosophila in various molecular and cellular contexts. We found that while loss of either Gr32a or Gr66a abolishes sensitivity to lobeline (LOB), berberine (BER), and denatonium (DEN) in all labellar sensilla types, mutation of either Gr22e or Gr59c selectively impairs the detection of these chemicals in the S-b or I-a sensilla, respectively. Misexpression of either GR32a/GR59c/GR66a or GR22e/GR32a/GR66a confers sensitivity to LOB, BER, and DEN on sweet GRNs and Drosophila S2 cells. We also found Gr22e expression in Gr59c mutant GRNs and Gr59c expression in Gr22e mutant GRNs rescues their detection of LOB, BER, and DEN. This suggests these two Grs are functionally redundant except for the additional detection of strychnine (STR) by the GR22e/GR32a/GR66a complex. Overexpression or misexpression of either Gr22e or Gr59c confers hypersensitivity or novel responsiveness to their respective agonists. The Gr22e , Gr59c double mutant shows a more severe defect in LOB, BER, or DEN avoidance than either the Gr22e or Gr59c single mutant. This may reflect an underlying potential for the graded modulation of repulsion to aversive chemicals. We have found that the detection of the same bitter compounds can be accomplished in different bitter GRNs by distinct bitter GR complexes. Since it is the specific combination of GRs expressed by each bitter GRN that determines its response profile, we propose the heterogeneity of bitter Gr expression across bitter GRNs diversifies bitter coding and broadens the behavioral repertoire with which insects respond to their chemical environment. Minimal receptors for bitter compound detection Labellar sensilla fall into five distinct functional classes depending on their electrophysiological response profiles (Fig. 1a ) [3] . Of these, the I-a sensilla respond specifically to the aversive chemicals LOB, BER, and DEN (Fig. 1b ). The bitter GRNs in I-a sensilla express six Grs: Gr32a , Gr33a , Gr39a.a , Gr59c , Gr66a , and Gr89a (Fig. 1b ). We, therefore, asked whether these six GRs are sufficient to make functional LOB, BER, and DEN receptors, and if so, what the minimal GR components for LOB, BER, and DEN detection are. Since L-type sensilla do not respond to aversive chemicals [8] , they are a convenient cell type in which to measure the responsiveness to aversive compounds conferred by misexpression of bitter Gr candidates. 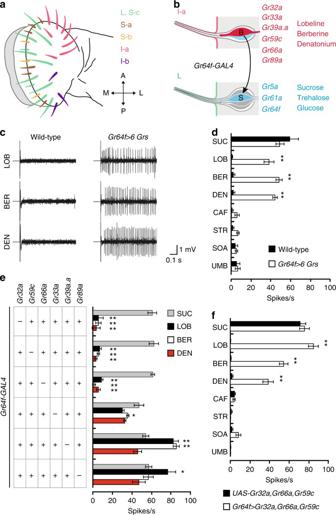To determine whether the combination of Gr32a , Gr33a , Gr39a.a , Gr59c , Gr66a , and Gr89a is sufficient for LOB, BER, and DEN detection, we misexpressed all six Grs in the sweet GRNs of L-type sensilla using Gr64f - GAL4 (Fig. Fig. 1 Identification ofGrsfor LOB, BER, and DEN detection.aSpatial localization of each class of taste bristle in the labellum. Figure modified from Weiss et al.3(2011).bSchematic for the misexpression of bitterGrsfrom I-a sensilla in the sweet GRNs of L-type sensilla usingGr64f-GAL4. TheGrsnormally expressed in bitter GRNs of I-a sensilla and their bitter ligands (red), as well as the sweetGrsnormally expressed in sweet GRNs of L-type sensilla and their sugar ligands (blue) are indicated.cRepresentative traces from L-type sensilla of flies of the indicated genotypes upon application of 1 mM stimuli of LOB, BER, or DEN.dMean responses of L-type sensilla induced by the indicated chemicals: 100 mM sucrose (SUC), 1 mM LOB, 1 mM BER, 1 mM DEN, 5 mM CAF, 1 mM STR, 1 mM SOA, and 1 mM UMB.n= 6–10. Unpairedt-test or the Mann−WhitneyU-tests as appropriate.eIdentification of theGrsrequired for LOB, BER, and DEN detection. The mean responses of L-type sensilla of the indicated genotypes upon application of 1 mM stimuli of LOB, BER, and DEN as well as 100 mM SUC are shown.n= 6–10. ANOVAs followed by Dunnet T3 post hoc tests for LOB and the Kruskal−Wallis tests followed by Mann−WhitneyUpost hoc tests for BER and DEN. The asterisks indicate statistically significant differences fromGr64f>6Grs flies ind.fThe mean responses of L-type sensilla expressingGr32a,Gr59c, andGr66ainduced by the indicated chemicals.n= 6–10. Unpaired Student’st-tests or the Mann−WhitneyU-tests as appropriate. All data are presented as means ± S.E.M. *p< 0.05, **p< 0.01. Complete genotypes are listed in Supplementary Table6 1b ) [22] and confirmed the misexpression of each Gr in the sweet GRNs by quantitative PCR (Supplementary Table 1 ). Importantly, control L-type sensilla respond only to sucrose, not to aversive chemicals (Fig. 1c, d ). Although misexpression of all six Grs in L-type sensilla has no effect on sucrose responses (Fig. 1d ), it confers robust responsiveness to LOB, BER, and DEN. Consistent with the response profile of I-a sensilla, misexpression of all six Grs in L-type sensilla does not confer responsiveness to caffeine (CAF), STR, sucrose octaacetate (SOA), or umbelliferone (UMB) (Fig. 1d ). In further validation of these results, we found L-type sweet GRNs co-expressing all six Grs respond to LOB, BER, and DEN in a dose-dependent manner (Supplementary Fig. 1a ). We next sought to identify which Grs are indispensable in the detection of LOB, BER, and DEN. To do so, we misexpressed in the sweet GRNs of L-type sensilla six groups of five Grs at a time, omitting one of the original six Grs per group. We found the absence of Gr32a , Gr59c , or Gr66a prevents ectopic responses to LOB, BER, and DEN, suggesting these three Grs are essential for LOB, BER, and DEN detection (Fig. 1e ). We next found misexpression of GR32a, GR59c, and GR66a together confers sensitivity to LOB, BER, and DEN (Fig. 1f ), but not CAF, STR, SOA, or UMB. This suggests GR32a/GR59c/GR66a together form a receptor for LOB, BER, and DEN. Since neither the expression of any one of these three Grs nor any combination of two of these three Grs (i.e., Gr32a / Gr66a , Gr32a / Gr59c , or Gr66a / Gr59c ) is sufficient to confer LOB, BER, and DEN sensitivity, GR32a, GR59c, and GR66a are the minimal and essential components for LOB, BER, and DEN detection (Supplementary Fig. 1b ). It is noteworthy that misexpression of Gr32a , Gr59c , and Gr66a did not affect the sucrose responses of sweet GRNs, even as it conferred LOB, BER, and DEN responses (Fig. 1d–f ). Furthermore, misexpression of Gr32a , Gr59c , and Gr66a in the sweet GRNs of a new Gr64 cluster deletion mutant ( Gr64af ) covering the coding regions of the entire Gr64 cluster conferred a similar level of sensitivity to LOB, BER, and DEN as that in wild-type sweet GRNs (Supplementary Figs. 1c , 2a ). Previous mutants of the Gr64 cluster either deleted additional neighboring genes or only deleted some genes of the cluster [22] , [23] , [24] , [25] , and were thus less suitable for this purpose. Loss of six of the nine sweet clade Grs does not affect ectopic responses to LOB, BER, and DEN upon Gr32a , Gr59c , and Gr66a expression in sweet GRNs. This indicates that the ectopic responses to LOB, BER, and DEN we observed are not due to erratic interactions between endogenous sweet clade GRs and misexpressed bitter GRs. I-a sensilla require Gr59c for bitter compound response None of the labellar sensilla of Gr32a and Gr66a mutant flies show a significant electrophysiological response to LOB, BER, or DEN (Supplementary Fig. 1d ) [15] . We asked whether loss of Gr59c also impairs sensitivity to LOB, BER, and DEN by generating a Gr59c mutant ( Gr59c 1 ) by ends-out homologous recombination (Supplementary Fig. 2f ) [26] . As expected, the I-a sensilla of Gr59c mutant flies do not respond to LOB, BER, or DEN (Fig. 2a, b ). The S-a and S-b sensilla of Gr59c 1 flies, which do not express Gr59c , show wild-type responses to LOB, BER, and DEN. This suggests other receptor complexes are responsible for LOB, BER, and DEN sensitivity in these sensilla (Fig. 2b ). In addition, we found Gr59c 1 flies show enhanced responses to CAF, STR, and UMB (Fig. 2b ). This is consistent with a previous report that the I-a sensilla of Gr59c mutant flies show increased sensitivity to CAF and UMB [21] . In addition to confirming this, we found loss of Gr59c also increases the sensitivity of S-a sensilla to STR and S-b sensilla to CAF. Fig. 2 Electrophysiological responses of Gr59c 1 mutant sensilla to bitter chemicals. a Representative traces from I5 sensilla from wild-type and Gr59c 1 flies upon application of 1 mM stimulations with the indicated chemicals. b Mean responses of the indicated sensilla in wild-type and Gr59c 1 flies to 1 mM stimuli of the indicated bitter compounds except 5 mM CAF. n = 6–50. Unpaired Student t -tests or Mann−Whitney U -tests as appropriate. All data are presented as means ± S.E.M. ** p < 0.01 Full size image Identifying Grs for bitter compound sensing in S-b sensilla S-b sensilla detect LOB, BER, and DEN in the absence of Gr59c , suggesting another GR complex recognizes these compounds in these sensilla. We, therefore, set out to identify the bitter Grs required for LOB, BER, and DEN detection in S-b sensilla. Bitter GRNs in S-b sensilla express 16 different Grs [3] . While Gr32a , Gr33a , and Gr66a are required for the detection of LOB, BER, and DEN [15] , [19] , Gr8a is not [14] . To investigate the rest of these 16 Grs , we obtained three Gr mutants that cover five Grs (i.e., Gr22e , Gr28b.a , Gr28b.d , Gr28b.e , Gr36c ) [27] and then generated five more mutants (i.e., Gr22f 1 , Gr28a 1 , Gr36a 1 , Gr39b 1 , Gr89a 1 ) by ends-out homologous recombination (Supplementary Fig. 2 ) [26] . We then examined the responses of their S-b sensilla to LOB, BER, and DEN. We were forced to exclude Gr39a.a and Gr59a ; the Gr39a.a mutant is adult-lethal, and our attempts at obtaining a Gr59a mutant were unsuccessful. Consistent with previous reports [15] , [19] , loss of Gr32a , Gr33a , or Gr66a nearly abolishes LOB, BER, and DEN-evoked action potentials in S-b sensilla (Fig. 3a–c ). In addition, we found the S-b sensilla of Gr22e mutant flies show significantly reduced responses to LOB, BER, and DEN (Fig. 3a–d ), whereas those of Gr22f and Gr39b mutants show selectively reduced responses to DEN (Fig. 3c ). Fig. 3 Identification of Grs for LOB, BER, and DEN detection in S-b sensilla. a – c Screening to identify the Grs required for the responses in S-b sensilla to LOB a , BER b , and DEN c . 1 mM of each chemical was used. n = 8–31. ANOVAs with Tukey or Dunnett T3 post hoc tests or Kruskal−Wallis tests with Mann−Whitney U post hoc tests as appropriate. The asterisks indicate statistically significant differences from wild-type flies. d Representative traces from wild-type and Gr22e 1 S5 sensilla upon application of LOB, BER, and DEN. e Mean responses of the indicated sensilla from wild-type and Gr22e 1 flies to 1 mM stimulations with the indicated bitter substances except 5 mM CAF. n = 6–30. Unpaired Student’s t -tests or Mann−Whitney U -tests as appropriate. f Mean responses of Gr32a , Gr66a , and Gr22e -expressing L-type sensilla induced by 1 mM stimulations with the indicated chemicals except 100 mM SUC and 5 mM CAF. n = 7–14. Unpaired Student’s t -tests or Mann−Whitney U -tests as appropriate. All data are presented as means ± S.E.M. * p < 0.05, ** p < 0.01. Complete genotypes are listed in Supplementary Table 6 Full size image S-b sensilla required Gr22e for bitter compound response Next, we sought a more detailed picture of the role Gr22e plays in the detection of aversive compounds. In addition to their reduced sensitivity to LOB, BER, and DEN, Gr22e mutant S-b sensilla show lower sensitivity to STR and SOA (Fig. 3e ). Gr22e mutant S-a sensilla are less sensitive to DEN and STR (Fig. 3e ). Since S-b sensilla lacking Gr22e show reduced responses to LOB, BER, DEN, STR, and SOA, we asked whether GR22e, together with GR32a and GR66a, forms the functional receptor for these bitter compounds. Misexpression of Gr22e , Gr32a , and Gr66a using Gr64f - GAL4 does not alter sucrose responses but it does confer sensitivity to LOB, BER, DEN, and STR on the sweet GRNs of L-type sensilla (Fig. 3f ). We also found ectopic co-expression of Gr22e , Gr32a , and Gr66a in sweet GRNs lacking the Gr64 cluster ( Gr64af ) confers sensitivity to LOB, BER, DEN, and STR, indicating GR22e/GR32a/GR66a represents the minimal complex necessary for LOB, BER, DEN, and STR responses (Supplementary Fig. 3a ). Since loss of Gr22f and Gr39b reduces the responses of S-b sensilla to DEN, we also asked whether Gr22f and Gr39b participate in the DEN receptor. Similar misexpression of either Gr22f or Gr39b with both Gr32a and Gr66a does not confer DEN sensitivity on the sweet GRNs of L-type sensilla (Supplementary Fig. 3b ). This suggests the reduced responses to DEN in the Gr22f and Gr39b mutants are non-specific. They may instead be due to the formation of a DEN-detecting complex with other GRs or to an indirect reduction in DEN responses. Gr22e and Gr59c are redundant in bitter compound detection Since Gr59c and Gr22e are expressed in different sensilla and independently participate in receptor complexes that each respond to LOB, BER, and DEN, we wondered whether Gr22e can substitute for Gr59c in I-a sensilla and vice versa in S-b sensilla. We, therefore, expressed wild-type Gr22e or Gr59c in bitter GRNs of Gr22e mutants using Gr33a-GAL4 . As expected, Gr22e expression rescues the Gr22e mutant phenotype in S-b sensilla (Fig. 4a–d ). In addition, Gr22e and Gr59c expression both induce hypersensitivity to LOB, BER, and DEN in S-a and S-b sensilla (Fig. 4a–c ). Only Gr22e , however, rescues the STR detection defect of Gr22e 1 S-b sensilla and induces STR hypersensitivity in S-a sensilla (Fig. 4d ). This suggests the GR22e/GR32a/GR66a complex detects STR, but the GR59c/GR32a/GR66a complex does not. Neither misexpression of Gr22e nor overexpression of Gr59c affects sensitivity to LOB, BER, and DEN in I-a sensilla (Fig. 4a–c ), but misexpression of Gr22e results in a novel response to STR in I-a sensilla (Fig. 4d ). Misexpression of Gr22e or Gr59c in I-b sensilla results in a novel response to LOB, BER, and DEN and misexpression of Gr22e also results in a novel response to STR in I-b sensilla (Fig. 4a–d ). Fig. 4 Functional redundancy of Gr22e and Gr59c . Mean responses in flies of the indicated genotypes evoked by 1 mM stimulations with LOB a , e , BER b , f , DEN c , g , or STR d , h . n = 6–69. ANOVAs followed by Tukey or Dunnett T3 post hoc tests or Kruskal−Wallis tests followed by Mann−Whitney U post hoc tests as appropriate. All data are presented as means ± S.E.M. The asterisks indicate statistically significant differences (* p < 0.05, ** p < 0.01) from wild-type flies. Complete genotypes are listed in Supplementary Table 6 Full size image Next, we expressed either wild-type Gr22e or Gr59c in bitter GRNs of Gr59c mutants using Gr33a-GAL4 . Misexpression of Gr22e or Gr59c in the S-a and S-b sensilla of Gr59c mutant flies leads to their hypersensitivity to LOB, BER, and DEN (Fig. 4e–g ). Expression of either Gr22e or Gr59c can rescue the defect in LOB, BER, and DEN sensitivity observed in the I-a sensilla of Gr59c mutants (Fig. 4e–g ). Misexpression of Gr22e or Gr59c in I-b sensilla results in a novel response to LOB, BER, and DEN (Fig. 4e–g ). Only Gr22e overexpression induces STR hypersensitivity in S-a and S-b sensilla and only Gr22e misexpression induces novel responses to STR in I-a and I-b sensilla (Fig. 4h ). In summary, expression of Gr22e in the Gr22e mutant and expression of Gr59c in the Gr59c mutant both rescue their respective mutant phenotypes, confirming the respective defects are attributable to loss of Gr22e or Gr59c . In addition, expression of Gr22e in the Gr59c mutant and Gr59c in the Gr22e mutant produce nearly identical responses to LOB, BER, and DEN. This indicates Gr22e can substitute for Gr59c and vice versa, except in the detection of STR. Conferring bitter chemical-induced currents on S2 cells To determine whether Gr22e and Gr59c are ion conducting subunits that confer bitter compound sensitivity, we co-expressed Gr22e , Gr32a , and Gr66a or Gr32a , Gr59c , and Gr66a in Drosophila S2 cells and performed whole-cell voltage-clamp recordings. Consistent with our in vivo gain-of-function results, we found both Gr combinations confer sensitivity to LOB, BER, and DEN on S2 cells (Supplementary Fig. 4 ). These novel responses, which appear as outwardly rectifying currents in Supplementary Fig. 4 , also seem to be dose-dependent. GR22e/GR32a/GR66a-expressing S2 cells also respond to STR, but neither GR22e/GR32a/GR66a-expressing S2 cells nor GR59c/GR32a/GR66a-expressing S2 cells respond to CAF or SOA (Supplementary Fig. 4e, j ). These results are consistent with our in vivo loss-of-function and misexpression results. Bitter compound detection in Gr22e Gr59c double mutants The S-a sensilla of both Gr22e and Gr59c single mutants show normal responses to LOB, BER, and DEN (Figs. 2 , 3 ). We initially assumed this was a result of the functional redundancy of Gr22e and Gr59c in the detection of LOB, BER, and DEN in the S-a sensilla. To test this possibility, we generated the Gr22e , Gr59c double mutant. When we measured the responses of the S-a sensilla to LOB, BER, and DEN, we found the S-a sensilla in the Gr22e , Gr59c double mutant does not show a significant reduction in response to LOB, BER, and DEN compared to the wild-type or single mutant with the exception of the comparison between the Gr22e , Gr59c double mutant and the Gr59c mutant in response to LOB (Fig. 5a ). We were particularly surprised to note that while Gr22e mutant S-a sensilla show reduced responses to DEN, those of the Gr22e , Gr59c double mutant do not (Fig. 5a ). These results suggest other Grs must play a role in the detection of LOB, BER, and DEN in S-a sensilla. Fig. 5 Effect of Gr22e and Gr59c mutation on S-a sensilla. Mean response of S-a sensilla of the indicated genotype to 1 mM stimulations with LOB a , BER b , and DEN c . n = 6–54. ANOVAs followed by Tukey or Dunnett T3 post hoc tests or Kruskal−Wallis tests followed by Mann−Whitney U post hoc tests as appropriate. All data are presented as means ± S.E.M. The asterisks indicate statistically significant differences (* p < 0.05, ** p < 0.01) Full size image Next, we measured the LOB, BER, and DEN sensitivity of the S-b and I-a sensilla of the Gr22e , Gr59c double mutants. We found Gr22e , Gr59c double mutant S-b sensilla show reduced sensitivity to LOB, BER, and DEN like Gr22e single mutant S-b sensilla, but their defect in LOB and DEN detection is not as severe (Fig. 5b ). Gr22e , Gr59c double mutant I-a sensilla, like those of the Gr59c single mutant, do not respond to LOB, BER, or DEN (Fig. 5c ). Differential contribution of labellar sensilla to avoidance Finally, we used a two-way choice assay to ask how the different types of labellar bitter-responsive sensilla contribute to feeding decisions. We gave flies a choice between 1 mM sucrose and 5 mM sucrose combined with different concentrations of aversive compounds (LOB, BER, and DEN). While wild-type flies demonstrate dose-dependent repulsion to all the bitter compounds we tested (Fig. 6 ), both Gr22e and Gr59c single mutant flies show reduced repulsion to LOB- or DEN-containing foods (Fig. 6a, c ). This defect is even more severe in the Gr22e , Gr59c double mutant (Fig. 6a, c ). These data indicate the respective contributions of the S-b and I-a sensilla to behavioral LOB and DEN aversion are independent and additive. Surprisingly, we found that while the Gr59c mutant demonstrates a significant defect in BER avoidance, the Gr22e mutant does not (Fig. 6b ). The Gr22e , Gr59c double mutant, however, shows an even more severe defect in BER avoidance than the Gr59c single mutant (Fig. 6b ). These data further suggest the gustatory system uses different types of sensilla expressing different receptors to direct subtly different behavioral responses depending on the bitter compound in question. Fig. 6 The contribution of Gr22e and Gr59c to bitter food aversion. Two-way choice assays using the indicated concentrations of a LOB, b BER, and c DEN. n = 4–12. ANOVAs followed by Tukey post hoc tests or Kruskal−Wallis tests followed by Mann−Whitney U post hoc tests as appropriate. All data are presented as means ± S.E.M. The asterisks and sharps indicate statistically significant differences from wild-type flies (* p < 0.05, ** p < 0.01) and from both Gr22e 1 and Gr59c 1 ( # p < 0.05, ## p < 0.01), respectively Full size image Here we have clarified several principles that inform our understanding of the Drosophila Grs that detect aversive compounds. First, three Grs seem to cooperate to form functional bitter compound receptors. We have shown in sweet GRNs and Drosophila S2 cells that co-expression of Gr22e , Gr32a , and Gr66a is sufficient to confer sensitivity to LOB, BER, DEN, and STR, while co-expression of Gr32a , Gr59c , and Gr66a confers sensitivity to LOB, BER, and DEN. This is reminiscent of our identification of the heterotrimeric L-canavanine receptor—GR8a, GR66a, and GR98b [20] . If we arrange these bitter GR complex components in decreasing order of tuning breadth from broad to narrow, the resulting order would be: Gr66a , Gr32a , Gr22e , and Gr59c . Second, although Drosophila GR complexes function as heteromultimers, they seem to remain promiscuous. A given GR complex can be activated by multiple bitter chemicals: GR22e/GR32a/GR66a by LOB, BER, DEN, and STR; GR32a/GR59c/GR66a by LOB, BER, and DEN. Conversely, the same bitter chemicals can activate several different Gr complexes. For example, BER activates GR22e/GR32a/GR66a, GR32a/GR59c/GR66a, and another unknown GR complex in S-a sensilla. Finally, different GRNs use distinct GR combinations even for detecting the same chemicals. S-b sensilla require GR22e/GR32a/GR66a to detect LOB, BER, and DEN, while I-a sensilla require GR32a/GR59c/GR66a to accomplish the same thing. Since the S-a sensilla of Gr22e , Gr59c double mutants remain sensitive to LOB, BER, and DEN, they must have at least one additional receptor complex for these aversive compounds. It is likely S-b sensilla also have another receptor complex that responds to LOB, BER, and DEN, because S-b sensilla in the Gr22e mutant still respond weakly to these chemicals and the S-b sensilla of Gr22e , Gr59c double mutants are more sensitive to these chemicals than those of the Gr22e single mutant, presumably due to increase of expression of unknown LOB, BER, and DEN receptor complexes in the Gr22e , Gr59c double mutants (Fig. 5b ). The fact that Gr22e , Gr59c double mutant S-a sensilla show a near wild-type response to LOB, BER, and DEN (Fig. 5 ) makes it clear that distinct bitter GR complexes (even in the same GRN) can detect overlapping sets of bitter compounds. What advantage does such a strategy provide? We speculate that this permits specific sensilla to fine tune their responses to bitter compounds. For example, increasing the expression of Gr22e in S-a or S-b sensilla would make them more sensitive to LOB, BER, DEN, and STR. As expected with such a scheme, loss of either Gr22e or Gr59c results in a partial impairment of LOB, BER, and DEN avoidance rather than a complete loss of aversion (Fig. 6 ). Although we could not exclude the possibility that the behavioral consequences of the loss of Gr22e or Gr59c were influenced by taste organs other than the labellum (e.g., the tarsal taste sensilla) (Fig. 6 ), this is unlikely because the Gr22e and Gr59c reporters are not expressed in the tarsal taste sensilla [28] . This raises the interesting possibility that distinct GR complexes sense bitter chemicals not only depending on the taste sensilla in which they are expressed but also the different taste organs. A growing body of evidence suggests interactions between Grs co-expressed in bitter GRNs are an important determiner of the GRN’s response profile [3] , [21] . We found overexpression or misexpression of Gr22e or Gr59c in S-a and S-b sensilla increases the endogenous response to LOB, BER, and DEN (Fig. 4 ). It is likely the extra GR22e or GR59c proteins bind GR32a and GR66a. This would form more LOB, BER, and DEN receptor complexes, increasing the sensitivity of the response to these chemicals. In contrast, neither misexpression of Gr22e nor overexpression of Gr59c affects LOB, BER, and DEN responses in I-a sensilla. Misexpression of Gr22e or overexpression of Gr59c in the Gr59c mutant results in a complete wild-type level rescue. It is possible that in wild-type I-a sensilla, most GR32a and GR66a molecules are already bound to GR59c, and therefore extra GR22e or GR59c do not form additional LOB, BER, and DEN receptors with GR32a and GR66a. Since misexpression of Gr22e or Gr59c in I-b sensilla confers on them novel sensitivity to LOB, BER, and DEN, it is possible the exogenous GR22e or GR59c proteins are out-competing other GRs for binding to the endogenous GR32a and GR66a molecules, forming novel LOB, BER, and DEN receptor complexes. If this hypothesis is true, we should see a concurrent reduction in the responses of these I-b sensilla to their normal ligands. Indeed, overexpression of Gr59c suppresses the normal I-b response to CAF, presumably secondary to a reduction in the number of functional CAF receptor complexes [3] , [21] . In addition, loss of Gr59c in I-a sensilla, which shifts their bitter response profile to one resembling that of I-b sensilla (Fig. 2b ) [21] , allows other GRs expressed in I-a sensilla to form new functional receptor complexes. This then alters their sensitivity to CAF, UMB, TPH, and other bitter compounds (Fig. 2b ) [21] . In summary, our results suggest bitter coding is much more complex and dynamic than expected. In the future, we hope to correlate changes in Gr expression with changes in environmental conditions and internal physiological states to better understand the dynamics of this system and how they affect animal behavior. Fly stocks All fly stocks were maintained on standard cornmeal-molasses agar medium at 25 °C and 60% humidity under a 12 h/12 h light/dark cycle, respectively. 70 FLP ,70 I - SceI / CyO (BL6934), Gr28b mi (BL24190), and Gr36c mi (BL26596) were obtained from the Bloomington Drosophila Stock Center. Gr22e 1 (#140936) was obtained from the Kyoto Stock Center. To minimize genetic background artifacts, all mutant strains were outcrossed to w 1118 for five generations. ΔGr32a was a gift from Hubert Amrein. Gr64f - GAL4 and UAS - Gr59c were gifts from John Carlson. Gr33a 1 , Gr66a ex83 , UAS - Gr33a , UAS - Gr66a , and Gr33a - GAL4 were previously described [18] , [19] . Gr64af harboring the deletion of the whole Gr64 cluster will be described in a separate manuscript in detail (Supplementary Fig. 2a ). Generation of transgenic flies UAS - Gr22e , UAS - Gr22f , UAS - Gr32a , UAS - Gr39a.a , UAS - Gr39b , and UAS - Gr89a were generated. 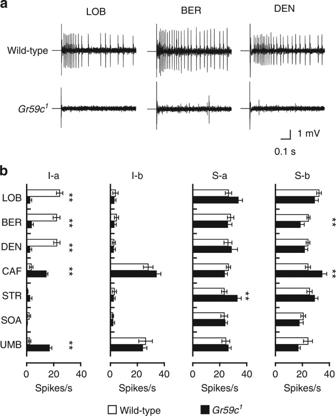Labellar cDNAs were synthesized using Thermo Scientific RevertAid Reverse Transcriptase (Thermo Fisher Scientific, Waltham, MA) followed by transcript extraction using TRIZOL (Thermo Fisher Scientific). Fig. 2 Electrophysiological responses ofGr59c1mutant sensilla to bitter chemicals.aRepresentative traces from I5 sensilla from wild-type andGr59c1flies upon application of 1 mM stimulations with the indicated chemicals.bMean responses of the indicated sensilla in wild-type andGr59c1flies to 1 mM stimuli of the indicated bitter compounds except 5 mM CAF.n= 6–50. Unpaired Studentt-tests or Mann−WhitneyU-tests as appropriate. All data are presented as means ± S.E.M. **p< 0.01 Individual Gr cDNAs were amplified and cloned from total labellar cDNAs using primer pairs listed in Supplementary Table 2 . The amplified DNA fragments were inserted into pUAST vectors via conventional molecular cloning methods. pUAST vectors carrying each Gr cDNA were injected into w 1118 embryos by standard transgenesis techniques (BestGene Inc., Chino Hills, CA). 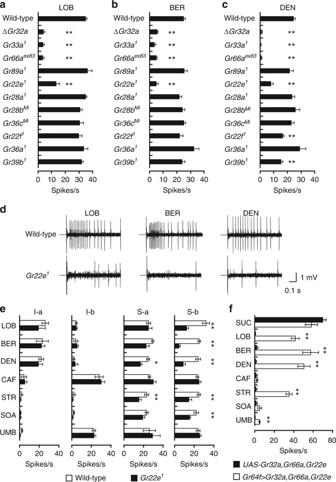Generation of Gr mutants Gr22f 1 , Gr28a 1 , Gr36a 1 , Gr39b 1 , Gr59c 1 , and Gr89a 1 were generated by homologous recombination [26] . Fig. 3 Identification ofGrsfor LOB, BER, and DEN detection in S-b sensilla.a–cScreening to identify theGrsrequired for the responses in S-b sensilla to LOBa, BERb, and DENc. 1 mM of each chemical was used.n= 8–31. ANOVAs with Tukey or Dunnett T3 post hoc tests or Kruskal−Wallis tests with Mann−WhitneyUpost hoc tests as appropriate. The asterisks indicate statistically significant differences from wild-type flies.dRepresentative traces from wild-type andGr22e1S5 sensilla upon application of LOB, BER, and DEN.eMean responses of the indicated sensilla from wild-type andGr22e1flies to 1 mM stimulations with the indicated bitter substances except 5 mM CAF.n= 6–30. Unpaired Student’st-tests or Mann−WhitneyU-tests as appropriate.fMean responses ofGr32a,Gr66a, andGr22e-expressing L-type sensilla induced by 1 mM stimulations with the indicated chemicals except 100 mM SUC and 5 mM CAF.n= 7–14. Unpaired Student’st-tests or Mann−WhitneyU-tests as appropriate. All data are presented as means ± S.E.M. *p< 0.05, **p< 0.01. Complete genotypes are listed in Supplementary Table6 In general, 3 kb 5′ and 3′ homology arms for each Gr coding region were amplified by genomic DNA PCR using primer pairs listed in Supplementary Table 3 and cloned into mutant construction vectors. pw35 was used for Gr22f 1 , Gr36a 1 , Gr39b 1 , and Gr89a 1 . pw35 GAL4 and pw35 + were used for Gr28a 1 and Gr59c 1 , respectively. After obtaining transformants carrying each targeting vector, the transgenes were mobilized by crossing to 70 FLP ,70 I - SceI / CyO . 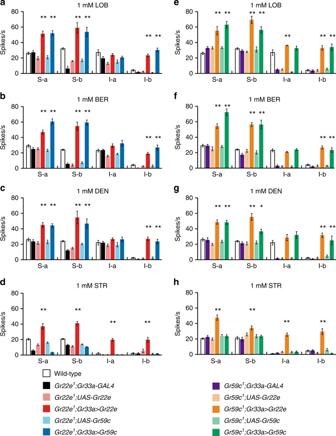Mosaic-eyed progeny (F1) were crossed to w 1118 to obtain red-eyed F2 progenies, which were subjected to PCR analysis [29] . Fig. 4 Functional redundancy ofGr22eandGr59c. Mean responses in flies of the indicated genotypes evoked by 1 mM stimulations with LOBa,e, BERb,f, DENc,g, or STRd,h.n= 6–69. ANOVAs followed by Tukey or Dunnett T3 post hoc tests or Kruskal−Wallis tests followed by Mann−WhitneyUpost hoc tests as appropriate. All data are presented as means ± S.E.M. The asterisks indicate statistically significant differences (*p< 0.05, **p< 0.01) from wild-type flies. Complete genotypes are listed in Supplementary Table6 Each Gr mutation was confirmed by genomic PCR using primers listed in Supplemental Table 4 . Quantitative PCR Total RNA was extracted from dissected labella using TRIZOL (Thermo Fisher Scientific) according to the manufacturer’s instructions. Labellar cDNA was synthesized from 1 μg of total RNA with the RevertAid reverse transcriptase system (Thermo Fisher Scientific). Quantitative PCR was conducted with a Quantstudio3 real-time PCR instrument (Thermo Fisher Scientific) using the ABI SYBR green system (Applied Biosystems, Foster City, CA). 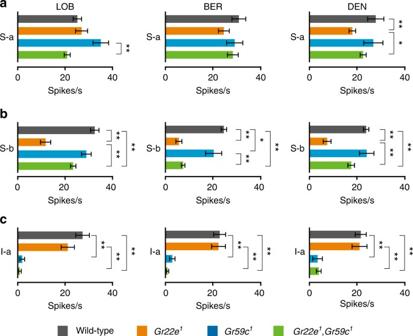C T values were measured in triplicate. Fig. 5 Effect ofGr22eandGr59cmutation on S-a sensilla. Mean response of S-a sensilla of the indicated genotype to 1 mM stimulations with LOBa, BERb, and DENc.n= 6–54. ANOVAs followed by Tukey or Dunnett T3 post hoc tests or Kruskal−Wallis tests followed by Mann−WhitneyUpost hoc tests as appropriate. All data are presented as means ± S.E.M. The asterisks indicate statistically significant differences (*p< 0.05, **p< 0.01) The sequence of the primer pairs for each Gr are shown in Supplementary Table 5 . The concentrations of the linearized DNA carrying each of 6 Grs were measured with a Nanodrop (Thermo Fisher Scientific) and a series of 10-fold dilutions of linearized DNA were subjected to quantitative PCR analysis to establish standard curves and determine their regression equation. The average C T value for each target gene obtained from the same genotype were then used to calculate the absolute copy numbers for each Gr transcript in labella of the indicated genotypes. Absolute copy number of the target gene \(= \left( {{\mathrm{copy}}\,{\mathrm{number}}\,{\mathrm{of}}\,{\mathrm{the}}\,{\mathrm{standard}}} \right) \times 10^{\left( {{\mathrm{Ct}} - {\mathrm{b}}} \right)/{\mathrm{m}}}\) , where b and m refer to the slope and intercept of the standard curve regression equation, respectively. The number of transcripts in sweet GRNs was calculated by subtracting the number of transcripts in the Gr64f - GAL4 control (endogenous bitter Gr expression level) from the number of transcripts of flies ectopically expressing Grs . RNA extraction and quantitative PCR were performed at least three times. Tip recording 2–5-day-old flies housed in fresh vials were anesthetized by brief ice exposure. A glass capillary pipette containing Ringer’s solution was inserted through the thorax to the base of the labellum and connected to ground to serve as the reference electrode. The indicated concentrations of each tastant compound were dissolved in 30 mM tricholine citrate for electrical conductivity in a 10–20 μm diameter recording electrode. After the recording electrode was connected to a TastePROBE (Syntech, Hilversum, The Netherlands), the electrical signals derived from taste sensilla were recorded using an acquisition controller (Syntech) attached to a computer. These signals were amplified (×10), band-pass-filtered (100–3000 Hz), and sampled at 12 kHZ. Neuronal firing rates were then analyzed using the Autospike 3.1 software (Syntech). Two-way choice behavioral assay Briefly, 40–50 3–5-day-old flies were collected under CO 2 anesthesia at least 1 day prior to starvation. The flies were starved for 18 h in vials containing only 1% agarose gel. Then, they were given 90 min in a dark room at room temperature to choose between 1% agarose gel containing 1 mM sucrose or 5 mM sucrose and the indicated concentrations of bitter chemicals. To monitor their food preference, each food was mixed with either a blue (0.125 mg/ml Brilliant blue FCF) or red (0.2 mg/ml sulforhodamine B) non-toxic dye. After freezing the flies, the color of their abdomens was scored under a stereomicroscope. A preference index was calculated using the following equation: Preference Index (PI) = (# of red or blue abdomens + ½ the # of purple abdomens)/Total # of fed flies. Whole-cell patch clamp recordings Gr - and EGFP-expressing S2 cells on coverslips were transferred to a chamber positioned on the stage of an inverted microscope (IX73, Olympus, Tokyo, Japan). Whole-cell currents were measured using a multiclamp amplifier at a holding potential of –60 mV (Axon Instruments, Foster City, CA) at room temperature. The bath solution contained normal Ringer’s solution: 140 mM NaCl, 5 mM KCl, 2 mM CaCl 2 , 2 mM MgCl 2 , 10 mM HEPES (titrated to pH 7.4 with NaOH). The pipette solution contained 140 mM CsCl, 5 mM EGTA, 10 mM HEPES, 2 mM MgATP, 0.2 mM NaGTP (titrated to pH 7.2 with CsOH). Electrodes were pulled from borosilicate glass to a final resistance of 2–4 MΩ after fire-polishing. The seal resistances were 3–10 GΩ. After establishing a whole-cell configuration, currents were recorded in the presence of LOB, BER, DEN, CAF, STR, or SOA by applying 400 ms voltage-ramp pulses from −80 to +80 mV every 1500 ms. Currents were digitized with a Digidata 1440 A converter (Axon Instruments), filtered at 5 kHz, and analyzed using Clampfit 10.2 (Axon Instruments). Chemicals Berberine, caffeine, denatonium, lobeline, sucrose, sucrose octacetate, strychnine, sulforhodamine B, tricholine citrate, and umbelliferone were purchased from Sigma-Aldrich (Saint Louis, MO). Brilliant blue FCF was purchased from Wako Pure Chemical Industries, Ltd (Osaka, Japan). Statistics All data were subjected to the Levene and Kolmogrov−Smirnov tests to evaluate variance homogeneity and normality, respectively. Depending on the results of these tests, ANOVAs with Tukey or Dunnet T3 post hoc tests or Kruskal−Wallis tests with Mann−Whitney U post hoc tests were used to identify significant differences in comparisons between multiple groups. The unpaired Student’s t -test or the Mann−Whitney U -test was used for comparisons between two groups. Data availability All relevant data are available from the authors upon request.